Mitotic spindle orientation predicts outer radial glial cell generation in human neocortex The human neocortex is increased in size and complexity as compared with most other species. Neocortical expansion has recently been attributed to protracted neurogenesis by outer radial glial cells in the outer subventricular zone, a region present in humans but not in rodents. The mechanisms of human outer radial glial cell generation are unknown, but are proposed to involve division of ventricular radial glial cells; neural stem cells present in all developing mammals. Here we show that human ventricular radial glial cells produce outer radial glial cells and seed formation of the outer subventricular zone via horizontal divisions, which occur more frequently in humans than in rodents. We further find that outer radial glial cell mitotic behaviour is cell intrinsic, and that the basal fibre, inherited by outer radial glial cells after ventricular radial glial division, determines cleavage angle. Our results suggest that altered regulation of mitotic spindle orientation increased outer radial glial cell number, and ultimately neuronal number, during human brain evolution. The human neocortex has undergone a marked expansion as compared with other vertebrate species [1] , [2] . Recent studies have begun to uncover unique structural and cellular features of the fetal primate brain that may account for its increased size and neuronal number, but the underlying mechanisms are not yet clear [3] , [4] , [5] , [6] . While both the developing primate and rodent brains contain a ventricular zone populated by neural stem cells called ventricular radial glial (vRG) cells [7] , [8] , [9] , [10] , the primate neocortex displays an additional region of neurogenesis that is absent in rodents; the outer subventricular zone (oSVZ) [3] , [6] , [11] . The oSVZ is located at a distance from the ventricle and contains a large proportion of outer RG (oRG) cells, neural stem cells that express vRG markers but display important characteristics distinct from vRG cells. Both vRG and oRG cells maintain basal fibres that extend as far as the pial surface and function as guides for neuronal migration [10] , [12] , [13] , but only vRG cells display apical end feet that contact the ventricle and form adherens junctions with other vRG end feet [14] , [15] . Both vRG and oRG cells have the ability to self-renew and produce neurogenic intermediate progenitor (IP) cells, but mouse IP cells undergo only one round of division to produce two neurons [16] , [17] , while human IP cells undergo many transit-amplifying rounds of cell division before producing neurons [3] . Thus, oRG cells appear to contribute to human neocortical expansion by increasing the absolute number of neuronal progenitor cells, and by giving rise to more neuronal progeny per progenitor cell. What cellular mechanisms led to an expanded oRG cell population and oSVZ size in the developing human brain? Evolutionary changes in mitotic spindle orientation could have altered the way cell fate determinants are segregated during vRG cell mitosis, affecting daughter cell fate and function and possibly leading to increased oRG cell generation. In vRG cells, cell fate determinants initially identified in Drosophila melanogaster neuroblasts associate preferentially with the apical domain or basal fibre [1] , [18] , [19] . These structures are differentially inherited in vRG daughter cells that subsequently display asymmetric fates [20] . While localization of both progenitor [21] , [22] and neural [23] , [24] , [25] fate determinants has been demonstrated at the apical domain, inheritance of the basal domain and fibre has been hypothesized as important for maintaining stem cell identity [1] , [4] , [26] , [27] , [28] . In rodents, the majority of vRG divisions are oriented vertically, with a cleavage furrow perpendicular to the ventricular surface [27] , [29] , [30] , [31] , [32] , [33] , [34] , [35] . During neurogenesis, one daughter inherits the basal fibre and half of the apical domain, becoming a self-renewed vRG cell. The other daughter inherits half of the apical domain, delaminates during the next cell cycle, and adopts a neuronal or IP cell fate [16] , [31] . Interestingly, molecular perturbations that induce non-vertical cleavages in rodent vRG cells lead to the more basal daughter inheriting the basal fibre but no part of the apical domain, and adopting oRG-like morphology [31] . These experiments suggest a possible evolutionary mechanism for increasing oRG cell generation in the fetal human brain. During early brain development (before gestation week 10 (GW10)), the majority of vRG divisions in human cortex are vertically oriented [36] , but studies of mitotic spindle regulation later in development during oSVZ formation and oRG production have been extremely limited. We wanted to test whether regulation of mitotic spindle orientation is altered in fetal human neocortex during peak neurogenesis, when the oSVZ appears, and whether this leads to increased oRG cell production. Here, we show that oRG cells in the developing human cortex are produced from vRG cells following division with a non-vertical cleavage orientation in which the basal daughter inherits the basal fibre and becomes the new oRG cell. We further show that the vast majority of oRG divisions display a horizontal cleavage plane, leading to oRG cell self-renewal by the daughter that inherits the basal fibre. We observe that cell-intrinsic mechanisms establish cleavage angle and control mitotic somal translocation (MST) [3] , an oRG-specific mitotic behaviour, in oRG-like cells in dissociated culture. An increase in non-vertical divisions of vRG cells may have contributed to the evolutionary expansion of the human neocortex by allowing large numbers of oRG cells to be generated, greatly increasing the number of neural progenitor cells. Furthermore, the tight regulation of mitotic spindle orientation in both vRG and oRG division increases the ways by which neurogenesis could be affected in diseases that disrupt cleavage angle regulation, such as lissencephaly and microcephaly [2] , [37] , [38] , [39] , [40] , [41] . Horizontal vRG divisions produce oRG cells Expansion of the oRG cell population within the oSVZ coincides with peak neurogenesis in the developing human neocortex [3] ; however, the origin of oRG cells in humans is unknown. It was recently demonstrated that a very small population of oRG cells exists in the mouse and is generated from oblique divisions of vRG cells [31] , [42] . We hypothesized that human oRG cells are likewise generated from horizontal or oblique vRG cell divisions in which the newly generated oRG daughter inherits the basal fibre and no part of the apical membrane. We investigated this by performing time-lapse imaging of dividing vRG cells in GW16 through GW18 human cortical slices. We sparsely labelled cortical cells by infection with a CMV-GFP adenovirus (Adeno-GFP), and observed that vRG cells underwent interkinetic nuclear migration (INM) ( Supplementary Movie 1 ), as previously described in other species [16] . In contrast to the primarily vertically oriented divisions in mouse cortex, we observed a mix of divisions displaying vertical (60–90°), oblique (30–60°) and horizontal (0–30°) cleavage planes with respect to the ventricular surface. Of the 70 observed divisions at the ventricular surface, 21 were vertical, 6 were oblique and 43 were horizontal. While cell movement out of the imaging field and short imaging time windows sometimes precluded analysis of daughter cell fate after cell division, we observed 15 divisions that appeared to produce an oRG daughter cell as defined by rapid translocation away from the ventricular surface and maintenance of a basal fibre but no apical end foot ( Supplementary Movie 2 and Fig. 1a ). Nearly all (14/15) of these divisions were horizontal, while the remaining division was oblique. In seven of these oRG-generating divisions, we observed that the apical daughter clearly began to regrow a basal fibre, suggesting a self-renewed vRG fate. Finally, we performed fate staining on four pairs of daughter cells after horizontal division, and observed that in all cases, the daughter cell that adopted oRG morphology maintained Sox2 expression and did not express Tbr2, consistent with oRG and not IP cell fate, and the apical daughter cell was similarly Sox2+/Tbr2−, consistent with a self-renewed vRG fate ( Fig. 1b ). We concluded that non-vertical divisions produce oRG cells in fetal human cortex. 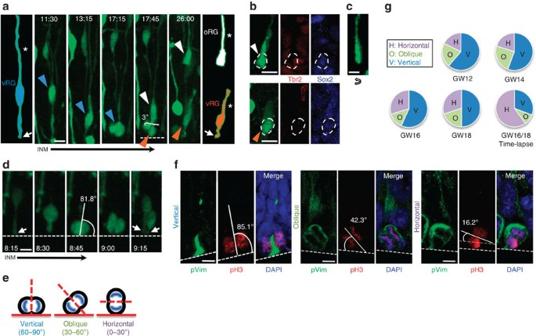Figure 1: Horizontal vRG divisions produce oRG cells. (a) Time-lapse stills of horizontal vRG division labelled with Adeno-GFP in GW16 human fetal cortical slice that results in generation of an oRG cell. vRG cell (blue arrowhead) starts at a distance from the ventricle, descends during INM, and divides with a horizontal spindle orientation at the ventricular surface (dotted white line at 17:45). Basal daughter (white arrowhead) retains basal fibre (asterisk) and rapidly exits the ventricular zone, adopting an oRG cell morphology. Apical daughter (orange arrowhead) inherits entire apical domain (white arrow) and regrows a basal fibre, becoming a self-renewed vRG cell. Cells of interest are schematized at beginning and end of sequence to more clearly demonstrate morphology and inheritance of basal fibre and apical domain. Scale bar, 10 μm. (b) Fate staining of daughter cells from division inaconfirms that the basal daughter (white arrowhead) is Tbr2−/Sox2+, consistent with oRG identity, and the apical daughter (orange arrowhead) is also Tbr2−/Sox2+, consistent with vRG identity. Scale bar, 10 μm. (c)z-plane analysis of basal daughter from division in panelarotated 90° confirms lack of apical process. Scale bar, 10 μm. (d) Time-lapse stills of vertical vRG division in GW16 human fetal cortical slice after which both daughters inherit half of the AD (white arrows) and neither daughter adopts oRG morphology. Part of the basal fibre is not visible due to its location out of the imagedz-stack. Scale bar, 10 μm. (e) Schematic of vRG cells undergoing mitosis at the ventricular surface (solid red line) with vertical, oblique and horizontal cleavage angles. Mitotic spindle orientation was analysed with respect to the ventricular surface. (f) Images of vRG cells in fixed human fetal cortical slices undergoing mitosis with vertical (left), oblique (center), and horizontal (right) mitotic spindle orientations at the ventricular surface. Scale bars, 5 μm. (g) Quantification of mitotic spindle orientation in fixed slices throughout peak neurogenesis and oRG cell generation, and during time-lapse imaging of GW16/18 human fetal cortical slices. Cells used for calculation in fixed slices were pH3+, pVim+ cells in anaphase or telophase that displayed a basal fibre and were located at the ventricular surface. Figure 1: Horizontal vRG divisions produce oRG cells. ( a ) Time-lapse stills of horizontal vRG division labelled with Adeno-GFP in GW16 human fetal cortical slice that results in generation of an oRG cell. vRG cell (blue arrowhead) starts at a distance from the ventricle, descends during INM, and divides with a horizontal spindle orientation at the ventricular surface (dotted white line at 17:45). Basal daughter (white arrowhead) retains basal fibre (asterisk) and rapidly exits the ventricular zone, adopting an oRG cell morphology. Apical daughter (orange arrowhead) inherits entire apical domain (white arrow) and regrows a basal fibre, becoming a self-renewed vRG cell. Cells of interest are schematized at beginning and end of sequence to more clearly demonstrate morphology and inheritance of basal fibre and apical domain. Scale bar, 10 μm. ( b ) Fate staining of daughter cells from division in a confirms that the basal daughter (white arrowhead) is Tbr2−/Sox2+, consistent with oRG identity, and the apical daughter (orange arrowhead) is also Tbr2−/Sox2+, consistent with vRG identity. Scale bar, 10 μm. ( c ) z -plane analysis of basal daughter from division in panel a rotated 90° confirms lack of apical process. Scale bar, 10 μm. ( d ) Time-lapse stills of vertical vRG division in GW16 human fetal cortical slice after which both daughters inherit half of the AD (white arrows) and neither daughter adopts oRG morphology. Part of the basal fibre is not visible due to its location out of the imaged z -stack. Scale bar, 10 μm. ( e ) Schematic of vRG cells undergoing mitosis at the ventricular surface (solid red line) with vertical, oblique and horizontal cleavage angles. Mitotic spindle orientation was analysed with respect to the ventricular surface. ( f ) Images of vRG cells in fixed human fetal cortical slices undergoing mitosis with vertical (left), oblique (center), and horizontal (right) mitotic spindle orientations at the ventricular surface. Scale bars, 5 μm. ( g ) Quantification of mitotic spindle orientation in fixed slices throughout peak neurogenesis and oRG cell generation, and during time-lapse imaging of GW16/18 human fetal cortical slices. Cells used for calculation in fixed slices were pH3+, pVim+ cells in anaphase or telophase that displayed a basal fibre and were located at the ventricular surface. Full size image During rodent neurogenesis, the majority of vRG cell divisions at the VZ have vertical cleavage planes, after which both daughters inherit half of the apical domain [31] . One daughter cell may subsequently delaminate from the VZ, presumably becoming a neuron or IP cell. We asked whether in human vRG cells, vertical cleavages also led to inheritance of a portion of the apical domain by both daughter cells. Similar to rodent cortex, in 100% (12/12) of vertical vRG divisions in which the apical domains were clearly visible before and after cell division, both daughter cells inherited a portion of the apical membrane ( Fig. 1d ). These results suggest that, in contrast to oblique and horizontal divisions, vertical vRG cell divisions do not produce oRG cell daughters. Instead, vertical divisions in humans may be similar to those in rodent cortex, resulting in one self-renewed vRG cell, and one IP cell or neuron that subsequently delaminates. Horizontal vRG divisions occur throughout oSVZ expansion We next examined regulation of vRG cell mitotic spindle orientation over time from GW12 to GW18, the period of peak neurogenesis in primate neocortex [1] , [6] . The oSVZ is expanding in size throughout this period, and oRG cells are increasing in number [3] . As our analysis showed that oRG cells are produced by non-vertical divisions, we predicted that we would observe horizontal and oblique vRG cleavages throughout this period. We performed immunohistochemistry on fixed GW12, 14, 16 and 18 human fetal neocortical tissue samples. We used an antibody against phosphorylated vimentin (pVim) to mark cells in M phase and to identify vRG cells by their ventricular location and basal fibre, co-staining with an antibody against phosphorylated histone H3 (pH3) to visualize chromosomes during mitosis. We then analysed mitotic spindle orientation of vRG cells in either anaphase or telophase at the VZ ( Fig. 1e ). We found a small increase in the percentage of horizontal/oblique divisions throughout this time period, from 37.5% at GW12 to 50% at GW18 ( n =35–60 cells total from at least five different sections, generated from at least two different tissue samples for each age) ( Fig. 1g ). Vertical divisions had a corresponding decrease, from 62.5% at GW12 to 50% at GW18. These observations represent an increased proportion of vertical divisions as compared with results from time-lapse imaging of dividing vRG cells at GW16/18, where 69.2% of divisions were horizontal/oblique and 30.8% were vertical, possibly reflecting the influence of cell culture conditions or a slight disruption of the ventricular surface in slice culture. Our observation that a much higher proportion of non-vertical vRG divisions occurs in humans than has been reported in rodents [29] , [30] , [31] , [32] , [33] , [34] , [35] , the large increase in oRG cells in humans as compared with rodents [3] , [42] , and the evidence we have presented here for the synchronous timing of non-vertical vRG divisions with oRG cell generation and oSVZ expansion [3] , further support a role for non-vertical vRG division in oRG cell generation. oRG cells divide horizontally to self-renew Our results indicated that during non-vertical vRG division, inheritance of the basal fibre and failure to inherit the apical domain coincide with oRG cell generation. It has been previously demonstrated that oRG divisions are self-renewing, where the more basal daughter maintains oRG identity, and the more apical daughter adopts either oRG or IP cell fate [3] . We asked whether oRG cells divide with a horizontal spindle orientation, thereby allowing the more basal cell to retain the oRG cell identity associated with the basal fibre. We first examined oRG cell divisions in organotypic slice culture, noting that cells underwent MST, a highly dynamic process during which the nucleus moves a distance of ~50 μm in the basal direction along the basal fibre within a 1-h period before cytokinesis [3] . oRG cell divisions generated a basal oRG daughter, and appeared horizontally oriented, with the cleavage plane perpendicular to the basal fibre ( Fig. 2a–c and Supplementary Movie 3 ). While oRG cells do not contact the ventricular surface, we nonetheless observed that 27.5% of oRG cells displayed short apical processes of mean length 8.4 μm ( Fig. 3a–d ). To determine how the spindle orientation of oRG divisions compared with vRG divisions, we quantified cleavage plane angles in fixed GW16 brain slices, identifying oRG cells in anaphase or telophase by their basal fibre, pVim reactivity and pH3 staining of condensed chromatin ( Fig. 2d ). This analysis revealed that the majority (96.3%) of oRG divisions were non-vertical (horizontal or oblique). A significantly higher proportion of oRG divisions were oriented horizontally (82.0%) when compared with vRG divisions at the ventricular surface (29.7%) (Pearson’s Chi-squared test, P <0.0005) ( Figs 1g and 2h ). Correspondingly, there were significantly fewer vertical oRG divisions (2.8%) as compared with vertical vRG divisions (56.8%) (Pearson’s Chi-squared test, P <0.0005). We concluded that horizontal spindle orientation is an actively regulated component of self-renewing oRG divisions. 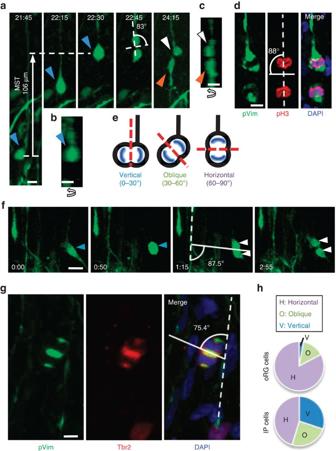Figure 2: oRG cells divide horizontally to self-renew. (a) Time-lapse stills of a dividing oRG cell (blue arrowhead) in GW16 human fetal cortical slice labelled with Adeno-GFP. The cell undergoes MST and divides with a horizontal spindle orientation, producing an apical daughter (orange arrowhead) and a basal daughter (white arrowhead). The basal daughter retains the basal fibre and becomes a self-renewed oRG cell, while the apical daughter produces an apical process. Scale bar, 10 μm. (b)z-plane analysis of oRG cell in first frame ofa, demonstrating lack of apical process. Scale bar, 10 μm. (c)z-plane analysis of daughter cells in last frame ofa, demonstrating lack of apical process on basal daughter, and presence of apical process on apical daughter. Scale bar, 10 μm. (d) Image of oRG cell in fixed GW16 human fetal cortical oSVZ undergoing mitosis with a horizontal cleavage plane. Scale bar, 10 μm. (e) Schematic of oRG cells undergoing mitosis with vertical, oblique and horizontal cleavage planes. Cleavage plane angle was analysed with respect to the basal fibre of the dividing cell (or in the case of IP cells, with respect to the nearest basal fibre). (f) Time-lapse stills of IP cell (blue arrowhead) in a GW18 human fetal cortical slice that retracts its processes and rounds up to divide symmetrically, without undergoing MST or INM, to produce two daughter cells (white arrowheads). Spindle orientation was calculated with respect to the nearest radial fibre. Scale bar, 20 μm. (g) Image of IP cell in fixed GW16 human fetal cortical oSVZ undergoing mitosis with a horizontal spindle orientation. Scale bar, 5 μm. (h) Quantification of mitotic spindle orientations in i/oSVZ progenitors (oRG cells and IP cells) in fixed GW16 human fetal cortical slices. Cells used for calculation were in anaphase or telophase and displayed the following characteristics; oRG cells: pVim+, pH3+ cells in the iSVZ or oSVZ that displayed a basal fibre but no apical ventricular contact; IP cells: Tbr2+ cells in the iSVZ or oSVZ that were pVim+ and displayed no basal or apical fibre. Figure 2: oRG cells divide horizontally to self-renew. ( a ) Time-lapse stills of a dividing oRG cell (blue arrowhead) in GW16 human fetal cortical slice labelled with Adeno-GFP. The cell undergoes MST and divides with a horizontal spindle orientation, producing an apical daughter (orange arrowhead) and a basal daughter (white arrowhead). The basal daughter retains the basal fibre and becomes a self-renewed oRG cell, while the apical daughter produces an apical process. Scale bar, 10 μm. ( b ) z -plane analysis of oRG cell in first frame of a , demonstrating lack of apical process. Scale bar, 10 μm. ( c ) z -plane analysis of daughter cells in last frame of a , demonstrating lack of apical process on basal daughter, and presence of apical process on apical daughter. Scale bar, 10 μm. ( d ) Image of oRG cell in fixed GW16 human fetal cortical oSVZ undergoing mitosis with a horizontal cleavage plane. Scale bar, 10 μm. ( e ) Schematic of oRG cells undergoing mitosis with vertical, oblique and horizontal cleavage planes. Cleavage plane angle was analysed with respect to the basal fibre of the dividing cell (or in the case of IP cells, with respect to the nearest basal fibre). ( f ) Time-lapse stills of IP cell (blue arrowhead) in a GW18 human fetal cortical slice that retracts its processes and rounds up to divide symmetrically, without undergoing MST or INM, to produce two daughter cells (white arrowheads). Spindle orientation was calculated with respect to the nearest radial fibre. Scale bar, 20 μm. ( g ) Image of IP cell in fixed GW16 human fetal cortical oSVZ undergoing mitosis with a horizontal spindle orientation. Scale bar, 5 μm. ( h ) Quantification of mitotic spindle orientations in i/oSVZ progenitors (oRG cells and IP cells) in fixed GW16 human fetal cortical slices. Cells used for calculation were in anaphase or telophase and displayed the following characteristics; oRG cells: pVim+, pH3+ cells in the iSVZ or oSVZ that displayed a basal fibre but no apical ventricular contact; IP cells: Tbr2+ cells in the iSVZ or oSVZ that were pVim+ and displayed no basal or apical fibre. 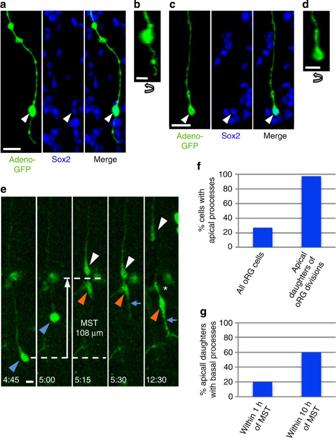Figure 3: Apical and basal processes on oRG cells and oRG apical daughters. (a) oRG cell with apical process in GW18 human fetal oSVZ, identified by morphology after 18-h Adeno-GFP infection followed by fixation and Sox2 staining. Scale bar, 20 μm. (b)z-plane analysis of cell in panelarotated 90° confirms the presence of apical process. Scale bar, 10 μm. (c) oRG cell lacking apical process in GW18 human fetal oSVZ, identified by morphology after Adeno-GFP infection and by Sox2 positivity. Scale bar, 20 μm. (d)z-plane analysis of cell in panelcrotated 90° confirms lack of apical process. Scale bar, 10 μm. (e) Time-lapse stills of a dividing oRG cell (blue arrowhead) in GW18 human fetal cortical slice labelled with Adeno-GFP. The oRG cell undergoes MST and produces an apical daughter (orange arrowhead) and a basal daughter (white arrowhead). The basal daughter retains the basal fibre and becomes a self-renewed oRG cell. The apical daughter produces an apical process immediately after MST (blue arrow), and a basal process several hours after MST (asterisk), adopting bipolar morphology. Scale bar, 10 μm. (f) Quantification of presence of apical process on all oRG cells in the GW16/18 human fetal i/oSVZ, and on apical daughters of oRG cell divisions after time-lapse imaging of GW16/18 human fetal cortex. All apical processes on apical daughters were produced within 1 h of MST. (g) Quantification of presence of basal process on apical daughters of oRG cell divisions after time-lapse imaging in GW16/18 human fetal cortex. Unlike the apical process, the basal process often takes more than 1 h to begin growing after MST. Full size image Figure 3: Apical and basal processes on oRG cells and oRG apical daughters. ( a ) oRG cell with apical process in GW18 human fetal oSVZ, identified by morphology after 18-h Adeno-GFP infection followed by fixation and Sox2 staining. Scale bar, 20 μm. ( b ) z -plane analysis of cell in panel a rotated 90° confirms the presence of apical process. Scale bar, 10 μm. ( c ) oRG cell lacking apical process in GW18 human fetal oSVZ, identified by morphology after Adeno-GFP infection and by Sox2 positivity. Scale bar, 20 μm. ( d ) z -plane analysis of cell in panel c rotated 90° confirms lack of apical process. Scale bar, 10 μm. ( e ) Time-lapse stills of a dividing oRG cell (blue arrowhead) in GW18 human fetal cortical slice labelled with Adeno-GFP. The oRG cell undergoes MST and produces an apical daughter (orange arrowhead) and a basal daughter (white arrowhead). The basal daughter retains the basal fibre and becomes a self-renewed oRG cell. The apical daughter produces an apical process immediately after MST (blue arrow), and a basal process several hours after MST (asterisk), adopting bipolar morphology. Scale bar, 10 μm. ( f ) Quantification of presence of apical process on all oRG cells in the GW16/18 human fetal i/oSVZ, and on apical daughters of oRG cell divisions after time-lapse imaging of GW16/18 human fetal cortex. All apical processes on apical daughters were produced within 1 h of MST. ( g ) Quantification of presence of basal process on apical daughters of oRG cell divisions after time-lapse imaging in GW16/18 human fetal cortex. Unlike the apical process, the basal process often takes more than 1 h to begin growing after MST. Full size image The apical daughters of oRG cell divisions may adopt an oRG cell fate, or may become IP cells, expressing Tbr2 and undergoing further transit-amplifying divisions [3] . We characterized the morphology of apical oRG daughters, observing that in the majority of divisions (97.5%), the apical daughter produced an apical process within 1 h of MST, ( Fig. 3e ). Within 1 h, only 20% of apical daughters displayed a basal process, though this number increased to 60% within 10 h, after which no further cells were observed to grow a basal process ( Fig. 3e ). Thus, the majority of apical daughters of oRG division ultimately adopt a bipolar morphology, though it is not yet clear how this correlates with IP cell versus oRG cell fate. IP cells divide symmetrically with a random cleavage angle The predominantly horizontal divisions of oRG cells exploit the intrinsic polarity of these cells to asymmetrically segregate the basal fibre, potentially along with unidentified cell fate determinants, into the self-renewing oRG daughter. We hypothesized that mitotic spindle orientation would be randomly distributed in IP cells, which are morphologically symmetrical and produce daughter cells with symmetric fates [16] . In contrast to vRG and oRG cells, which undergo INM and MST, respectively, IP cells retract their processes, round up and divide in place ( Fig. 2f ). We quantified cleavage plane angles in GW16 cortex of IP cells in anaphase or telophase, using the nearest pVim+ radial fibre as a reference point, as the radial fibre scaffold is oriented perpendicularly to the ventricular surface [10] . IP cells were identified by their location in the iSVZ or oSVZ, positive Tbr2 staining, and a lack of basal fibre by pVim staining ( Fig. 2g ). Unlike oRG cells, which are located in the same region but undergo predominantly horizontal divisions, IP cell cleavage angles appeared randomly distributed ( Fig. 2h ). Thus, it appears as though the molecular machinery that controls mitotic spindle orientation and basal fibre inheritance in oRG cells is not active in IP cells. Horizontal divisions are cell-intrinsic in oRG-like cells In the developing rodent cortex, contact with the pial surface does not appear necessary for vRG function [43] . However, it is unknown whether oRG cell function requires signals from surrounding brain structures, such as through oRG cell basal process contact with the basal lamina or blood vessels. To determine whether MST and its associated horizontal spindle orientation required extrinsic directional cues or would persist outside of the native cortical environment, we dissociated fetal human neocortex, labelled cells using Adeno-GFP, and performed time-lapse imaging for up to 10 days. We found that 19% of cells displayed one process analogous to the basal process of oRG cells, 29% displayed two processes, 48% were multipolar and 4% did not display any processes ( Supplementary Fig. S1 ). The ‘two-process' group likely also contained oRG cells, as 27% of oRG cells in vivo display a short apical process ( Fig. 3f ). In dissociated cortical progenitor cell cultures generated from two different ages of samples (GW14 and GW16), we observed that MST occurred in cells displaying one prominent process with or without a second, smaller process ( Fig. 4a ). As MST appears to be an identifying behaviour of oRG cells, which has not been shown to occur in any other cell type in the developing brain, we called progenitor cells in culture that displayed MST ‘oRG-like cells’. oRG-like divisions contrasted with symmetric, IP-like divisions, which were far more numerous and in which cells rounded up and divided in place ( Fig. 4b ). While we occasionally observed oscillatory behaviour of bipolar cells reminiscent of INM ( Supplementary Movie 4 ), we did not observe any unambiguous examples of INM. Furthermore, INM is defined based on the direction of cell movement with respect to structures extrinsic to the cell, such as the ventricular surface or adhesion belt, and our dissociated cultures lacked epithelial features that would normally be present in vivo , in slice cultures or in neural rosettes. Thus, we were able to further investigate MST, but not INM, in dissociated cell culture. 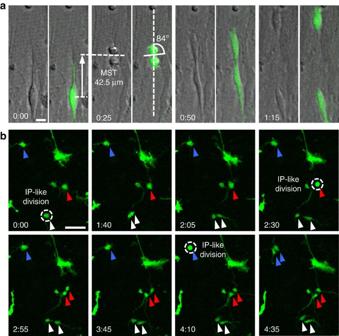Figure 4: Dissociated cortical progenitor cells display MST and horizontal spindle orientation. (a) oRG-like cell in dissociated culture undergoes MST followed by division with horizontal cleavage angle. Dissociated cortical cells were infected with low-titre GFP adenovirus or retrovirus and grown in culture for up to 5 weeks. Transmitted light microscopy allowed visualization of condensed chromatin for quantification of spindle orientation. Scale bar, 10 μm. (b) Multiple IP-like cell divisions in culture, which contrast with oRG-like divisions by their lack of MST. Individual multipolar cells were followed (blue, red and white arrowheads), and over a period of less than 5 h, each cell underwent mitosis (dotted circle) without MST, producing two multipolar daughter cells. Scale bar, 50 μm. Figure 4: Dissociated cortical progenitor cells display MST and horizontal spindle orientation. ( a ) oRG-like cell in dissociated culture undergoes MST followed by division with horizontal cleavage angle. Dissociated cortical cells were infected with low-titre GFP adenovirus or retrovirus and grown in culture for up to 5 weeks. Transmitted light microscopy allowed visualization of condensed chromatin for quantification of spindle orientation. Scale bar, 10 μm. ( b ) Multiple IP-like cell divisions in culture, which contrast with oRG-like divisions by their lack of MST. Individual multipolar cells were followed (blue, red and white arrowheads), and over a period of less than 5 h, each cell underwent mitosis (dotted circle) without MST, producing two multipolar daughter cells. Scale bar, 50 μm. Full size image We next wanted to determine how closely MST in dissociated culture resembled the observations in slice culture. The majority of oRG-like divisions (85.7%) had a ‘horizontal’ cleavage angle, or orthogonal with respect to the basal fibre orientation ( Fig. 5a ). The mean MST distance was 72.6 μm, similar to published observations of MST in oRG cells in slice culture [3] ( Fig. 5b ). Several oRG-like cells were observed to undergo divisions in which the daughter cell that did not inherit the basal fibre grew a basal fibre during the next cell cycle, adopting an oRG-like morphology and subsequently undergoing MST and dividing ( Supplementary Movie 5 and Fig. 5c ). This corresponds to observations in slice culture, in which the more apical daughter after an oRG division may grow a new basal fibre, thereby expanding the oRG population [3] . In some cases, daughter cells translocated in directions that were independent of the original direction of MST, and depended only on the location of the newly grown ‘basal’ fibre. We concluded that MST and horizontal cleavage plane orientation, progenitor cell behaviours unique to oRG cells, persist outside of the native context of the developing neocortex. MST appears to be a cell-intrinsic process, and the basal fibre directs establishment of a horizontal spindle orientation. MST may require signalling factors, such as mitogens from neighbouring cells, but does not require a radial fibre scaffold or cues derived from contact with the basal lamina, blood vessels or meninges. 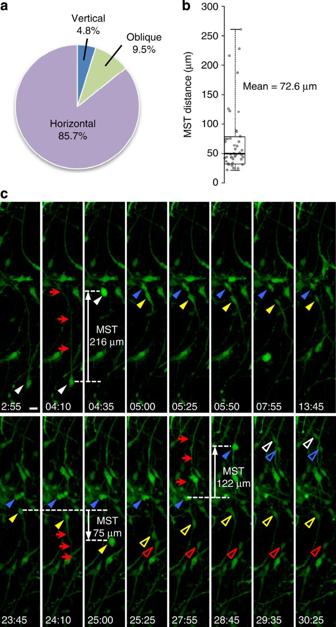Figure 5: MST and establishment of a horizontal spindle orientation are cell-intrinsic processes. (a) Quantification of cleavage angles in oRG-like cells in dissociated culture in which transmitted light microscopy allowed visualization of spindle orientation. (b) Box plot of MST distances for oRG-like divisions in dissociated culture. (c) Time-lapse stills of dissociated, Adeno-GFP-labelled GW16 human neocortical progenitor cell divisions. oRG-like cell (white arrowhead) with basal process (red arrows) undergoes MST along the basal process and divides at 4:35 to produce two daughter cells: a ‘basal’ daughter (blue arrowhead) and an ‘apical’ daughter (yellow arrowhead). The apical daughter grows a basal fibre (red arrows) in the opposite direction as the original basal fibre, and subsequently undergoes MST in the direction of the newly generated fibre at 25:00 to produce two daughter cells (open yellow arrowhead, open red arrowhead). The basal daughter of the first division extends its basal fibre (red arrows) in the same orientation as the original basal fibre, and undergoes MST in the direction of this fibre. This cell divides at 28:45 to produce two daughter cells (open white arrowhead, open blue arrowhead). Scale bar, 20 μm. Figure 5: MST and establishment of a horizontal spindle orientation are cell-intrinsic processes. ( a ) Quantification of cleavage angles in oRG-like cells in dissociated culture in which transmitted light microscopy allowed visualization of spindle orientation. ( b ) Box plot of MST distances for oRG-like divisions in dissociated culture. ( c ) Time-lapse stills of dissociated, Adeno-GFP-labelled GW16 human neocortical progenitor cell divisions. oRG-like cell (white arrowhead) with basal process (red arrows) undergoes MST along the basal process and divides at 4:35 to produce two daughter cells: a ‘basal’ daughter (blue arrowhead) and an ‘apical’ daughter (yellow arrowhead). The apical daughter grows a basal fibre (red arrows) in the opposite direction as the original basal fibre, and subsequently undergoes MST in the direction of the newly generated fibre at 25:00 to produce two daughter cells (open yellow arrowhead, open red arrowhead). The basal daughter of the first division extends its basal fibre (red arrows) in the same orientation as the original basal fibre, and undergoes MST in the direction of this fibre. This cell divides at 28:45 to produce two daughter cells (open white arrowhead, open blue arrowhead). Scale bar, 20 μm. Full size image We present here a model by which horizontal divisions may have contributed to the evolutionary expansion of the human neocortex by increasing oRG cells and their neuronally committed progeny ( Fig. 6 ). We show that during peak neurogenesis in human cortex, between 37.5% and 50% of vRG cell divisions have a non-vertical (horizontal or oblique) cleavage plane, leading to the more basal daughter inheriting the basal fibre but not the apical end foot and adopting an oRG cell fate. This represents a large increase over the mouse, in which fewer than 10% of vRG divisions are non-vertical [27] , [29] , [30] , [31] , [32] , [33] , [34] , [35] . A recent study by Fietz et al . indicated that the majority of divisions at the ventricular surface of the fetal human brain display a vertical cleavage angle, but the authors did not take into account morphological criteria (presence of a basal fibre) to ensure that only vRG cells were analysed [4] . Other cell types, such as short neural precursors and IP cells, divide at the ventricular surface and may account for many of the vertical divisions observed in that study [32] , [44] , [45] , [46] . What mechanisms might have been responsible for an increase in horizontal vRG divisions in humans? Interestingly, expression of a dominant negative form of the spindle angle regulator LGN causes mouse vRG cells to display non-vertical cleavage angles and results in oRG-like cell production [31] . Mutations in LGN or other spindle angle regulators could have led to an increase in non-vertical vRG divisions in developing human cortex. It is also possible that other mechanisms of oRG cell generation exist, such as direct delamination, and we may have failed to observe this in our slice cultures due to a small sample size or our gestational age of analysis. 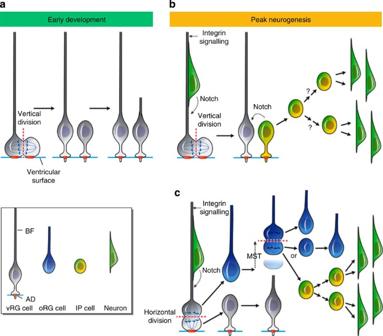Figure 6: Model of cleavage angle regulation of cell fate during human cortical development. (a) During early development, vRG divisions at the VZ are likely vertical, resulting in one daughter inheriting the basal fibre (BF), and both daughters inheriting half of the apical domain (AD) (orange). The daughter that retains the basal fibre maintains its apical contact and becomes a self-renewed vRG cell, whereas the daughter that does not receive the basal fibre likely also maintains its apical contact, generates a new basal fibre and adopts a vRG cell identity, thereby increasing the vRG progenitor population. (b) During peak neurogenesis, vRG divisions can either be vertical or horizontal/oblique. vRG division with vertical cleavage plane results in both daughter cells inheriting half of the AD. The cell that retains the basal fibre receives Notch and Integrin signalling via the basal fibre, maintains its apical contact and becomes a self-renewed vRG cell. The cell that does not inherit the basal fibre begins to express IP cell markers, including Notch ligands, thereby contributing to Notch activation of neighbouring vRG cells. The newly generated IP cell delaminates from the apical adhesion belt during the next cell cycle and migrates in a basal direction, where it may undergo multiple rounds of neurogenic divisions. (c) vRG division with a horizontal cleavage plane results in the more apical daughter inheriting the entire AD, regrowing a basal fibre, and becoming a self-renewed vRG cell. The more basal daughter inherits the basal fibre, rapidly exits the VZ and adopts an oRG cell fate. The newly generated oRG cell continues to divide horizontally, with the basal daughter inheriting the basal fibre and maintaining oRG cell identity. The apical daughter of horizontal oRG cell divisions either regrows a new fibre and adopts oRG cell fate, expanding the oRG cell population or becomes an IP cell and undergoes multiple rounds of neurogenic divisions. Figure 6: Model of cleavage angle regulation of cell fate during human cortical development. ( a ) During early development, vRG divisions at the VZ are likely vertical, resulting in one daughter inheriting the basal fibre (BF), and both daughters inheriting half of the apical domain (AD) (orange). The daughter that retains the basal fibre maintains its apical contact and becomes a self-renewed vRG cell, whereas the daughter that does not receive the basal fibre likely also maintains its apical contact, generates a new basal fibre and adopts a vRG cell identity, thereby increasing the vRG progenitor population. ( b ) During peak neurogenesis, vRG divisions can either be vertical or horizontal/oblique. vRG division with vertical cleavage plane results in both daughter cells inheriting half of the AD. The cell that retains the basal fibre receives Notch and Integrin signalling via the basal fibre, maintains its apical contact and becomes a self-renewed vRG cell. The cell that does not inherit the basal fibre begins to express IP cell markers, including Notch ligands, thereby contributing to Notch activation of neighbouring vRG cells. The newly generated IP cell delaminates from the apical adhesion belt during the next cell cycle and migrates in a basal direction, where it may undergo multiple rounds of neurogenic divisions. ( c ) vRG division with a horizontal cleavage plane results in the more apical daughter inheriting the entire AD, regrowing a basal fibre, and becoming a self-renewed vRG cell. The more basal daughter inherits the basal fibre, rapidly exits the VZ and adopts an oRG cell fate. The newly generated oRG cell continues to divide horizontally, with the basal daughter inheriting the basal fibre and maintaining oRG cell identity. The apical daughter of horizontal oRG cell divisions either regrows a new fibre and adopts oRG cell fate, expanding the oRG cell population or becomes an IP cell and undergoes multiple rounds of neurogenic divisions. Full size image In the oSVZ, we observed that 97.2% of oRG divisions were non-vertical, with more horizontal than oblique divisions, indicating active regulation of mitotic spindle orientation in oRG cells. In contrast, IP cell division appeared more random. Our results differ from those obtained by Fietz et al . [4] , who found that Pax6+ progenitors within the oSVZ display a random cleavage angle at GW14–16. However, they did not define oRG cells based on presence of a basal fibre as we did, which is important given co-expression in the P0 ferret i/oSVZ of Tbr2 and Pax6 in ~38% of progenitor cells [47] . We show here that in human fetal cortex, basal fibre inheritance is associated with oRG fate after horizontal vRG division, and oRG self-renewal after horizontal oRG division. Furthermore, oRG-like cells in dissociated culture undergo MST and maintain a horizontal cleavage plane during division. These observations suggest that the basal fibre could both orient oRG cell division and control stem cell function, possibly due in part to Integrin, Notch and/or retinoic acid signalling through the basal fibre [3] , [4] , [27] , [48] , [49] . The direction of MST in dissociated cultures was dependent on the orientation of the basal fibre, but not on the direction of MST in previous divisions. Therefore, secreted molecules or signals, such as those mentioned above from the glia, the basal lamina, the adjacent radial fibre scaffold or other sources may direct the prolonged growth of newly generated oRG and vRG basal fibres in situ , and prevent prolonged growth of apical processes, so that MST normally proceeds in the basal direction. The role of the apical domain is less clear than that of the basal fibre. Within the oSVZ, oRG cells do not express apical proteins found in vRG cells that are associated with retained stem cell function, such as Par3, ZO-1 or Prominin-1( [4] ). Similarly, we observed that after horizontal or oblique vRG divisions, the daughter that adopted oRG cell morphology did not inherit the apical domain. As oRG cells are able to produce neurogenic IP cells [3] , inheritance of the apical domain is not required for maintenance of neurogenic ability. The apical domain and adhesion belt appear to have a tethering role, allowing vRG cells to receive signals carried in the cerebrospinal fluid, maintaining the VZ as a neurogenic niche distinct from the i/oSVZ, and possibly directing vRG-specific behaviours, such as INM. We did not observe obvious INM in our dissociated cortical cultures, which may reflect the absence of an adherens junction belt present in vivo , in slices and at least partially in cultured neural rosettes [50] . It is possible that vRG cells that would have undergone INM were converted into oRG cells in dissociated culture due to lack of apical tethering, and therefore displayed MST as a result of basal-fibre mediated signalling. A previous study showed that loss of NUMB in mouse vRG cells leads to delamination and displacement from the ventricular zone due to disruption of adherens junctions, but that a progenitor state is nevertheless maintained [51] . This further supports a tethering role for the apical domain, and it is possible that the delaminated vRG cells either retained vRG identity or adopted oRG identity. Recent studies have demonstrated the presence of oRG cells and an oSVZ in agoutis (gyrencephalic rodents), and in marmosets, which are near-lissencephalic primates [52] , [53] , [54] , indicating that oRG cells are necessary, but not sufficient, for a gyrencephalic brain. Contributing mechanisms could include an increase in the total number of oRG cell divisions dependent on the length of brain development, decreases in cell cycle length in neural progenitor cells in the fetal human brain, and further differences in regulation of mitotic spindle orientation. Additionally, while rodent IP cells divide one time to produce two neurons, human IP cells in the oSVZ undergo many rounds of division before producing neurons [3] , [55] , [56] , suggesting that cortical expansion may be further explained by the increased transit amplification of oRG-generated IP cells. Taken together, our experiments demonstrate that regulation of mitotic spindle orientation is a conserved mechanism across species and cell types in the developing brain for controlling the balance of progenitor cell and neuronal populations. In vRG cells specifically, an increase in horizontal divisions may have contributed to neocortical expansion and gyrification in species such as humans that display an oSVZ and a large oRG cell population. Fetal tissue collection Fetal brain tissue was collected from elective pregnancy termination specimens at the San Francisco General Hospital, usually within 2 h of the procedure. Gestational age was determined using fetal foot length. Brain tissue was transported in L-15 medium on ice to the laboratory for further processing. Tissues were collected only with previous patient consent and in strict observance of legal and institutional ethical regulations. Research protocols were approved by the Gamete, Embryo and Stem Cell Research Committee (institutional review board) at the University of California, San Francisco. Imaging and cleavage angle analysis Brain tissue was fixed in 4% paraformaldehyde in PBS at 4 °C for 3 days, dehydrated in 30% sucrose in PBS, embedded and frozen at −80 °C in O.C.T. compound (Tissue-Tek), sectioned on a Leica CM3050S (50 or 20 μm) and stored at −80 °C. Cryosections were subjected to heat/citrate-based antigen retrieval for 10 min and permeabilized and blocked for 3–4 h in PBS plus 0.1% Triton X-100, 10% serum, 0.2% gelatin. Primary incubations were performed at 4 °C overnight. Washes and secondary incubations were standard procedures. Images were acquired on a Leica TCS SP5 broadband laser confocal microscope. Composite images were automatically stitched on acquisition using ‘Tilescan’ mode of Leica software. Images with morphological information are maximum intensity projections collected with at least 1-μm z -step size. Mitotic spindle orientations of cells in anaphase or telophase were measured using Screen Protractor (Iconico). The cleavage plane angle was calculated by determining the angle between the equatorial plate and the ventricular surface (vRG cells), the basal fibre (oRG cells) or the nearest basal fibre (IP cells). For quantification, vRG cells were defined as pVim+ cells at the ventricular surface with a basal fibre, oRG cells were defined as pVim+ cells in the iSVZ or oSVZ with a basal fibre but no apical ventricular contact (end foot), and IP cells were defined as pVim+ cells in the iSVZ or oSVZ that were Tbr2+ and displayed no basal or apical process. All proportions were calculated from between 35 and 60 cells in at least five different sections for each age generated from at least two different tissue samples for each age. Primary antibodies were: goat anti-SOX2 (Santa Cruz Biotechnology sc-17320, 1:250), rabbit anti-TBR2 (Millipore AB9618 or Abcam ab23345, 1:400), mouse anti-phospho-vimentin (MBL International D076-3S (Ser 55), 1:500), chicken anti-GFP (Aves Labs GFP-1020, 1:1,000), rabbit anti-phospho-histone-H3 (Abcam ab1791, 1:500), rabbit anti-nestin (Abcam ab5968, 1:200) and rabbit anti-PAX6 (Covance PRB-278P, 1:200). Secondary antibodies were: AlexaFluor 488 (1:1,000), 546 (1:500), 568 (1:500), 594 (1:500) or 647 (1:500)-conjugated donkey anti-goat, -rabbit or -mouse IgG or goat anti-chicken IgY (Invitrogen). Viral infection of slice culture and real-time imaging For time-lapse imaging experiments, brain tissue was transferred to an ice-chilled artificial cerebrospinal fluid (125 mM NaCl, 2.5 mM KCl, 1 mM MgCl 2 , 2 mM CaCl 2 , 1.25 mM NaH 2 PO 4 , 25 mM NaHCO 3 , 25 mM D -(+)-glucose, bubbled with 95% O 2 /5% CO 2 ), and blocks of cortical tissue were trimmed and imbedded in 4% low-melting-point agarose in artificial cerebrospinal fluid. Vibratome slices of 250–300 μm were generated and transferred to and suspended on Millicell-CM slice culture inserts (Millipore) in cortical slice culture medium, containing 66% Eagle's basal medium (BME), 25% Hanks, 5% FBS, 1% N-2, 1% penicillin, streptomycin and glutamine (all Invitrogen) and 0.66% D -(+)-glucose (Sigma). CMV-GFP adenovirus (Vector Biolabs, 1 × 10 6 colony-forming units (c.f.u.)) was directly applied to slices, and slices were cultured at 37 °C, 5% CO 2 , 8% O 2 for ~24 h, as described previously [3] . Cultures were then transferred to an inverted Leica TCS SP5 with an on-stage incubator (while streaming 5% CO 2 , 5% O 2 , balanced N 2 into the chamber) and imaged using a × 10 or × 40 air objective at 15–25-min intervals for up to 6 days with intermittent repositioning of the focal planes. Maximum intensity projections of the collected stacks (~30 μm at ~2.5-μm step size) were compiled and generated into movies, which were analysed using Imaris. Cleavage angle analysis was performed in a similar manner as for fixed tissue, using only divisions in which the cleavage furrow from anaphase through telophase was clearly visible. Quantification of vRG divisions in slices was performed on two or more slices each from n =5 individual tissue samples aged GW16–18. A total of 70 vRG cell divisions were analysed. Daughter cell morphology could not be definitively determined in all cases because imaging sessions could only last ~24 h due to subsequent distortion of the ventricular surface in vitro , and because in some cases, cells moved outside of the field of imaging. Because of these issues, analysis of the daughter cell fate after vRG division was performed on 31 pairs of daughter cells out of the 70 total pairs of daughter cells. Dissociated cortical progenitor culture and real-time imaging GW14–16 cortex was separated from meninges and cut into small pieces using a razor blade. Cells were dissociated by incubation with papain (Worthington Biochemical Corporation) at 37 °C for 20 min followed by addition of DNAse I and trituration. Dissociated cells were plated at a density of 250,000 cells per well in 12-well cell culture plates (Greiner Bio-one) pre-coated with matrigel (BD Biosciences). Cultures were maintained for up to 5 weeks in a DMEM-based dissociated culture medium containing 1% N-2, 1% B-27 supplement, 1% penicillin, streptomycin and glutamine (all Invitrogen), sodium pyruvate (0.11 mg ml −1 ), 1 mM N -acetylcysteine, with or without 10 ng ml −1 hFGF. CMV-GFP adenovirus (Vector Biolabs, 1 × 10 6 c.f.u.) or replication-incompetent enhanced-GFP-expressing retrovirus (1 × 10 6 c.f.u.) were applied to cells, which were cultured at 37 °C, 5% CO 2 , 8% O 2 until cells began expressing GFP (~24–48 h). Cultures were then transferred to an inverted Leica TCS SP5 with an on-stage incubator (while streaming 5% CO 2 , 5% O 2 , balance N 2 into the chamber), and imaged in both the GFP and transmitted light channels using a × 10 objective at 35-min intervals for up to 10 days. Movies were analysed using Imaris. Cleavage angle analysis was performed in a similar manner as for fixed tissue, using only divisions in which the condensed chromatin in anaphase or telophase was visible by transmitted light. A total of 41 oRG-like divisions from n =2 dissociated tissue samples were analysed. To determine the proportions of cell morphologies within dissociated cultures, cells were labelled as described above, and all cells that were bright enough to discern morphology were counted in four random fields of ~770 × 770 μm. For each cell, process number was defined as one of four groups: 0 (no discernable process), 1, 2 or >2 (multipolar). The average of the four proportion calculations from each field was then calculated for each group. Quantification of apical and basal processes To determine the proportion of oRG cells that display apical processes, GW16–18 human fetal cortical slices were infected with Adeno-GFP, cultured as described above for 18 h, fixed and stained for GFP, Sox2 and nestin. Confocal imaging was performed using a × 63 objective and images were analysed using Imaris. A total of 51 cells were analysed, and only cells that displayed a basal fibre and were GFP+/Sox2+ were used for quantification of apical process presence and length. Additionally, all oRG cells used for quantification were determined to be nestin+. For the analysis of apical and basal processes in apical daughters of oRG division, time-lapse imaging of GW16–18 slices was performed as described above on at least two slices each from n =3 individual tissue samples, and movies were analysed using Imaris. Forty oRG cell divisions in total were analysed, with oRG cells defined on the basis of oRG morphology (presence of a basal fibre, lack of ventricular contact) and mode of division (MST). After MST, an apical daughter was determined to have an apical process if a ventricular-directed process of any length appeared in the next cell cycle. An apical daughter was determined to have a basal process if a pial-directed process of any length appeared in the next cell cycle. Statistics For all measurements of cleavage angle proportions in fixed cryosections, between 35 and 60 cells were analysed from at least five sections for each age and cell type quantified. Proportions were compared pairwise using a Pearson’s Chi-square test. How to cite this article : LaMonica, B. E. et al . Mitotic spindle orientation predicts outer radial glial cell generation in human neocortex. Nat. Commun. 4:1665 doi: 10.1038/ncomms2647 (2013).